Estimating the potential public health impact of seasonal malaria chemoprevention in African children Seasonal malaria chemoprevention, previously known as intermittent preventive treatment in children, is highly effective in areas with a short malaria transmission season. Here we assess seasonality in malaria incidence data and define a predictor of seasonality based on rainfall. We then use spatial rainfall, malaria endemicity and population data to identify areas likely to have highly seasonal malaria incidence, and estimate the population at risk and malaria burden in areas where seasonal malaria chemoprevention would be appropriate. We estimate that in areas suitable for seasonal malaria chemoprevention, there are 39 million children under 5 years of age, who experience 33.7 million malaria episodes and 152,000 childhood deaths from malaria each year. The majority of this burden occurs in the Sahelian or sub-Sahelian regions of Africa. Our data suggest that seasonal malaria chemoprevention has the potential to avert several million malaria cases and tens of thousands of childhood deaths each year if successfully delivered to the populations at risk. Child mortality remains unacceptably high in many countries in sub-Saharan Africa, with malaria being a major contributor to this burden. Current estimates of malaria morbidity in Africa range from 174 million to 271 million clinical cases each year [1] , [2] , resulting in 600,000 to 1.1 million deaths [1] , [3] . Although there are uncertainties and limitations attached to each of these estimates, the burden of malaria is clearly unacceptably high and new malaria control measures are urgently needed, particularly for African children under 5 years of age. A series of studies conducted in Sahelian and sub-Sahelian Africa have shown that seasonal malaria chemoprevention (SMC), previously known as intermittent preventive treatment of malaria in children (IPTc), is a promising tool for the control of malaria in areas where transmission of malaria is highly seasonal. A meta-analysis of SMC studies in which a therapeutic course of sulphadoxine-pyrimethamine plus amodiaquine (SP-AQ) was given once per month to children under the age of 5 years during the peak malaria transmission season showed an 83% (95% CI: 72%, 89%) reduction in the incidence of clinical attacks of malaria and a similar reduction in the incidence of severe malaria (77%; 95% CI: 45%, 90%) [4] . Similar findings were obtained in a recent Cochrane review of IPTc studies [5] . The SP-AQ combination used in most trials was safe. Current evidence is consistent with a reduction in all-cause mortality due to SMC but the confidence intervals are wide (A.L.W., unpublished results) [4] , [5] . Similar results have been obtained with other antimalarial combinations given on a monthly basis. Administration every 2 months has also been tried but was less effective [6] . High levels of coverage have been achieved using community health workers to administer SMC, and the intervention is highly cost effective [7] , [8] . In the majority of studies, three monthly administrations have been employed and, although longer periods of administration may be considered, the evidence in relation to feasibility of delivery, safety and efficacy of SMC relates primarily to administration over a 3-month period. The World Health Organization (WHO) convened a meeting of a Technical Expert Group in May 2011 to consider whether sufficient data had been gathered to recommend incorporation of SMC into the malaria control programmes of areas with highly seasonal transmission of malaria. Their positive recommendation was reviewed by a newly constituted WHO Malaria Policy Advisory Committee in February 2012. If SMC with SP-AQ is formally recommended as policy by the Malaria Policy Advisory Committee, implementation may begin in certain countries of the Sahel and sub-Sahel sometime in 2012. Malaria control programme managers will need to consider whether regions of their country are suitable for the implementation of SMC on the basis of the incidence of malaria and its seasonality in those regions. To assist policy makers and programme managers in making such decisions, we have identified the geographical areas where SMC is likely to be an appropriate and cost-effective intervention using data on the overall incidence and seasonality of malaria in different parts of sub-Saharan Africa. In this study, we show that there are two large areas of Africa likely to have both sufficient seasonality and sufficient malaria incidence for SMC to be both effective and cost-effective. In particular, the Sahelian and sub-Sahelian regions of Africa have a large population of children under 5 years of age at risk in areas where SMC with current antimalarials is likely to be highly efficacious, and where millions of malaria cases and tens of thousands of childhood deaths could potentially be prevented each year. Defining areas suitable for the implementation of SMC Fifty-six sites where monthly malaria incidence had been measured for 12 consecutive months were identified in 22 sub-Saharan African countries ( Supplementary Tables S1,2 ). Areas meeting seasonality definition B (60% of annual incidence within 4 consecutive months) were observed more frequently in the Sahel and sub-Sahel than in other parts of Africa. Definition B gave consistent results in sites where more than one type of malaria outcome had been recorded (for example, severe malaria and clinical malaria) or where information was available for several years. Definition C (50% of annual incidence in 4 months) was not stringent enough to identify SMC areas, as a large number of sites had this level of seasonality. Definition A (75% of annual incidence in 4 months) excluded several sites known to be highly seasonal, including sites in the Gambia and Senegal, suggesting that this definition is too strict. Definition B was, therefore, used for subsequent analyses. After inspection of site-specific rainfall patterns, the severe malaria data reported for one site were considered unreliable (seasonality in malaria incidence was much stronger than the seasonality in rainfall), and this site was excluded as an outlier; 55 sites were, therefore, available for analysis ( Supplementary Tables S1,2 ). The best predictor of sufficient seasonality for SMC according to definition B was >60% of the total annual rainfall within three consecutive months; this cutoff identified areas with incidence patterns suitable for SMC with a sensitivity of 95.0% and a specificity of 73.5% ( Fig. 1 ). 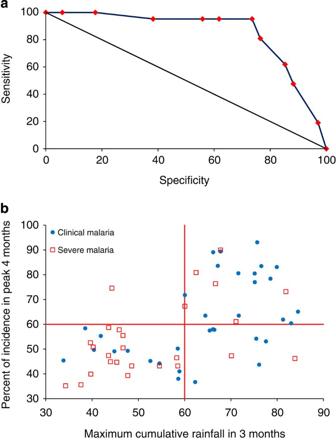Figure 1: Analysis of rainfall as a predictor of epidemiology suitable for SMC. (a) Receiver operating characteristic curve for binary indicator variables describing the percentage of the annual total rainfall occurring in 3 consecutive months. Dummy variables were created for 5% intervals between 0% and 100%. Observed values of cumulative rainfall in 3 months ranged from 33.8%–84.5%. The best indicator of SMC areas was rainfall greater than 60% in 3 months (sensitivity 95.0%, specificity of 73.5%). The black line indicates the reference line of no discrimination. (b) Maximum percentage of annual rainfall within 3 consecutive months compared with maximum percentage of malaria incidence within four consecutive months. The horizontal red line shows the cumulative incidence threshold within 4 months specified by definition B. The vertical red line shows discrimination of the data points by the best indicator based on rainfall (60% within 3 months). Figure 1: Analysis of rainfall as a predictor of epidemiology suitable for SMC. ( a ) Receiver operating characteristic curve for binary indicator variables describing the percentage of the annual total rainfall occurring in 3 consecutive months. Dummy variables were created for 5% intervals between 0% and 100%. Observed values of cumulative rainfall in 3 months ranged from 33.8%–84.5%. The best indicator of SMC areas was rainfall greater than 60% in 3 months (sensitivity 95.0%, specificity of 73.5%). The black line indicates the reference line of no discrimination. ( b ) Maximum percentage of annual rainfall within 3 consecutive months compared with maximum percentage of malaria incidence within four consecutive months. The horizontal red line shows the cumulative incidence threshold within 4 months specified by definition B. The vertical red line shows discrimination of the data points by the best indicator based on rainfall (60% within 3 months). Full size image Maps produced by rainfall seasonality alone, and by rainfall seasonality in areas endemic for Plasmodium falciparum , identified two broad areas as being potentially suitable for deployment of SMC ( Fig. 2a,b ). The first includes much of the Sahelian and sub-Sahelian regions of Africa, which matches well with the sites identified from the seasonality assessment of epidemiological data. The second area is in southern Africa, stretching from Namibia in the west to Mozambique and Southern Tanzania in the east. 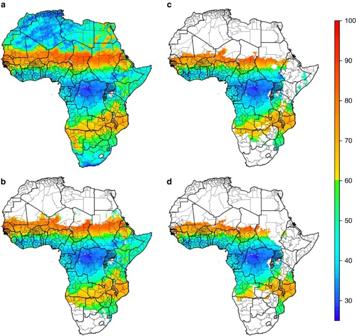Figure 2: Areas suitable for SMC implementation based on seasonality in rainfall and on malaria endemicity. (a). The maximum proportion of annual rainfall occurring within three consecutive months. Orange-red areas are those identified as suitable for SMC based on >60% of annual rainfall in 3 months. Green–blue areas indicate areas with less than 60% of annual rainfall within 3 months. First administrative level areas are superimposed on the map. (b) The maximum proportion of annual rainfall restricted to areas with stable endemicP. falciparum, as estimated by MAP21. (c) and (d) indicate rainfall seasonality in areas with prevalence above 8.8 and 17.3%, as estimated by MAP, corresponding to incidence above 0.1 and 0.2 cases per child per year, respectively. Figure 2: Areas suitable for SMC implementation based on seasonality in rainfall and on malaria endemicity. ( a ). The maximum proportion of annual rainfall occurring within three consecutive months. Orange-red areas are those identified as suitable for SMC based on >60% of annual rainfall in 3 months. Green–blue areas indicate areas with less than 60% of annual rainfall within 3 months. First administrative level areas are superimposed on the map. ( b ) The maximum proportion of annual rainfall restricted to areas with stable endemic P. falciparum , as estimated by MAP [21] . ( c ) and ( d ) indicate rainfall seasonality in areas with prevalence above 8.8 and 17.3%, as estimated by MAP, corresponding to incidence above 0.1 and 0.2 cases per child per year, respectively. Full size image Estimating the population and burden in SMC areas The geographical area mapped by rainfall seasonality, as defined above, in malaria endemic areas led to an estimate of 39 million children under 5 years of age at risk of malaria in areas suitable for implementation of SMC, 24.9 million in the Sahel or sub-Sahel and 14.1 million in southern and eastern Africa. On the basis of this population at risk, the method used in the World Malaria Report 2008 (WMR) [9] gave a total burden estimate of 33.7 million cases per year in children under 5 years of age in sites suitable for SMC, 24.1 million cases in the Sahel and sub-Sahel, and 9.6 million per year in the rest of Africa ( Table 1 ). The burden estimate using a prevalence-incidence relationship derived by the Malaria Atlas Project (MAP) [10] was 12 million malaria cases (see Methods ), 8.5 million of these in the Sahel and sub-Sahel. Mortality estimates using a fixed case fatality rate were 151,552 (108,506 in the Sahel and sub-Sahel) for the WMR burden estimate and 53,953 (38,474 in the Sahel and sub-Sahel) for the MAP burden estimate. Use of a population-based mortality rate, as described by Rowe et al . [11] gave an estimate of 314,283 deaths from malaria (221,811 in the Sahel and sub-Sahel). Applying a higher case fatality rate of 10 per 1,000 gave similar estimates to those produced using the method of Rowe et al . [11] (data not shown). Table 1 Estimated populations at risk, malaria incidence and malaria deaths in areas suitable for SMC. Full size table The burden in SMC areas above minimum incidence thresholds Applying lower prevalence thresholds to the map of areas suitable for SMC ( Fig. 2c,d ) produced smaller population estimates ( Tables 2 and 3 ): 28.9 million children under 5 years of age at risk in areas with incidence greater than 0.1 episodes per child during the transmission peak (21 million in the Sahel and sub-Sahel) and 24.9 million children at risk in areas with 0.2 episodes per child during the transmission peak (18.9 million in the Sahel and sub-Sahel). Corresponding morbidity and mortality estimates were slightly lower but remained substantial, particularly in the Sahel and sub-Sahel. The most stringent incidence threshold of 0.2 episodes per child during the transmission peak resulted in an estimate of 25.7 million malaria cases and 115,704 deaths (18.9 million cases and 85,225 deaths in the Sahel and sub-Sahel). Table 2 Impact of incidence thresholds on populations at risk and malaria burden estimates. 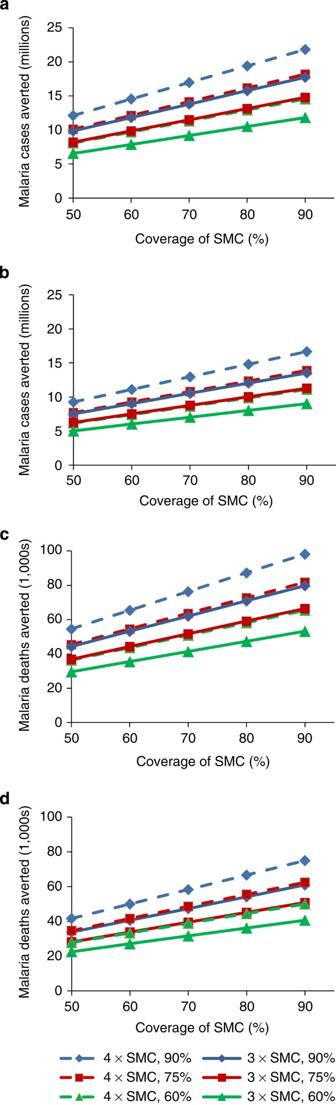Figure 3: Malaria cases and deaths potentially averted by SMC. Malaria cases and malaria deaths potentially averted in all areas suitable for SMC (a,c), and in areas with incidence >0.2 cases per child per year (b,d), with varying assumptions about efficacy, monthly coverage and the fraction of the burden occurring during the SMC period. 75% was considered the best estimate of the fraction of the total annual malaria burden occurring during the SMC period in SMC areas; 60 and 90% are also shown. Solid lines show impact for 3 SMC courses, assumed to have 65% efficacy as detailed in the text. Dotted lines show impact for 4 SMC courses, assumed to have 80% efficacy. The malaria burden estimate used for these calculations was that using the WMR method: 33,677,976 malaria cases in all SMC areas with stable endemicP.falciparum, and 25,712,319 derived from the population mapped by rainfall in areas with estimate of malaria incidence >0.2/child/year. Deaths refer to the constant-case fatality rate of 4.5 per 1,000, applied to the incidence estimates. Full size table Table 3 Impact of incidence thresholds on populations at risk and malaria burden estimates. Full size table Estimating the potential public health impact of SMC Using the WMR estimate of 33.7 million malaria cases per year in children under 5 years of age in the areas mapped as suitable for SMC, and 151,552 deaths per year (applying the fixed case fatality rate (CFR) to the incidence estimate), SMC is predicted to have a considerable impact ( Fig. 3 ). Restricting estimates to areas with incidence greater than 0.2 cases per child per year made only relatively minor changes. 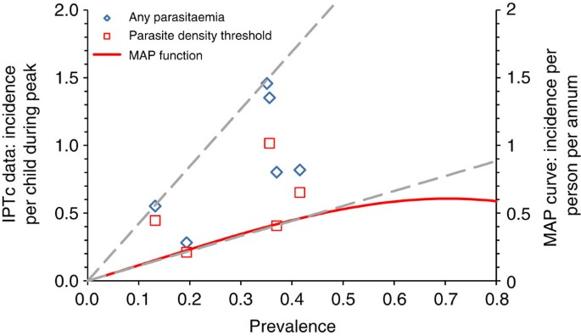Figure 4: Prevalence and incidence of malaria detected in SMC studies and the MAP prevalence-incidence relationship. Data points show observed incidence against end of season prevalence from control or placebo groups in IPTc studies from Niakhar, Senegal30; Hohoe, Ghana31; Kambila, Mali32; Bobo-Dioulasso, Burkina Faso (Zongo I., personal communication); Kati, Mali27and Boussé, Burkina Faso26. Data points show malaria incidence defined as fever plus parasitaemia of any density or with a local defined parasite density cutoff, and are shown against the left vertical axis. All studies included children under 5 years of age, with the exception of the Kambila IPTc study, which included children under 10 years of age. For the Kambila IPTc study (Mali) the prevalence estimate at the start of the transmission season (92/262, 35.1%) was used rather than that measured at the end of the transmission season, as this was based on relatively small numbers (8/54, 15%). The curve shows the fitted relationship between all age incidence per annum and prevalence in children 2–10 years of age, 13 and is shown against the right vertical axis. Dashed lines show the upper and lower limit of the incidence-prevalence relationship defined by the IPTc data points. Even if our approach has resulted in a 50% overestimate of the malaria burden in SMC areas, the potential impact of SMC could still be substantial, with ~5 million cases and 20,000 deaths averted if the intervention was widely deployed ( Table 4 ). Figure 3: Malaria cases and deaths potentially averted by SMC. Malaria cases and malaria deaths potentially averted in all areas suitable for SMC ( a , c ), and in areas with incidence >0.2 cases per child per year ( b , d ), with varying assumptions about efficacy, monthly coverage and the fraction of the burden occurring during the SMC period. 75% was considered the best estimate of the fraction of the total annual malaria burden occurring during the SMC period in SMC areas; 60 and 90% are also shown. Solid lines show impact for 3 SMC courses, assumed to have 65% efficacy as detailed in the text. Dotted lines show impact for 4 SMC courses, assumed to have 80% efficacy. The malaria burden estimate used for these calculations was that using the WMR method: 33,677,976 malaria cases in all SMC areas with stable endemic P . falciparum , and 25,712,319 derived from the population mapped by rainfall in areas with estimate of malaria incidence >0.2/child/year. Deaths refer to the constant-case fatality rate of 4.5 per 1,000, applied to the incidence estimates. Full size image Table 4 Sensitivity analysis of cases and deaths potentially averted by SMC. Full size table We have defined the epidemiological settings where SMC is likely to be a suitable intervention and mapped the geographical areas where this epidemiology is likely to be found. Climate-based predictors identified the highly seasonal areas suitable for SMC with high sensitivity and good specificity. It is clear from our estimates that there is a large population of children under 5 years of age at risk from malaria in areas where SMC is likely to be appropriate. The burden of malaria in these areas, particularly in countries in the Sahel and sub-Sahel, is substantial and suggests that SMC deployed at scale could have a major public health impact. Most evidence on the efficacy of SMC relates to delivery over 3 months. We chose to focus on incidence during a period of 4 consecutive months as this is the longest period for which 3 monthly courses of SMC might be expected to provide a reasonably high level of protection. Our assumption of impact during a 4-month peak was conservative as this was based on estimates of protective efficacy obtained from a study of children sleeping under insecticide treated nets over a three-and-a-half month follow-up period, assuming no protection in the subsequent two weeks. Although a considerable number of studies were identified in the literature review, only a small proportion of these reported morbidity data in the required format to assess seasonality in malaria burden reliably. Nevertheless, enough data points were found to explore the utility of different cutoffs to define malaria incidence as sufficiently seasonal for SMC to be valuable. As previously reported [12] , in sites with 2 rainy seasons, the largest number of cases per month did not necessarily occur in 4 consecutive months ( Supplementary Tables S1,2 ). Therefore, some situations where SMC may be appropriate, if directed at two seasonal peaks in transmission, may not have been identified by the approach used here. However, to date, SMC has not been used in such settings; whether this would be appropriate requires further investigation. Our approach focusses on epidemiological situations with a single peak in transmission, situations in which the efficacy of SMC has already been well characterized. Rainfall patterns delineated two distinct geographical areas where SMC could be considered. The estimates of populations of SMC areas defined in our analyses are consistent with the populations living in seasonal transmission areas determined by the Mapping Malaria Risk in Africa project [13] , but are more conservative ( Supplementary Tables S3,4 ). The map incorporating malaria endemicity is more biologically plausible than one based on rainfall alone as it excludes areas where rainfall may be seasonal but very low, or where other conditions prohibit malaria transmission. Malaria control programmes operating in countries bordering the area identified as being suitable for SMC should undertake assessment of the seasonality of malaria in these areas, using local incidence data to guide decisions about whether deployment of SMC would be appropriate. For example, rainfall in most of northern Ghana did not meet the seasonality criterion and our estimate of the population at risk in Ghana is consequently relatively small. However, the epidemiology of malaria in Navrongo, Ghana suggests that the northern regions may be suitable for SMC ( Supplementary Tables S1,2 ) [14] . Therefore, it is likely that a larger area could potentially benefit from SMC and a larger population could be protected than we have defined in this study. The continental maps showing areas suitable for SMC implementation covered primarily Sahelian and sub-Sahelian areas as expected a priori. Areas meeting the seasonality criterion were also found in southern and eastern Africa, where there is much less epidemiological information on the seasonality of malaria. In some of these areas, the incidence of malaria is low and unstable and therefore SMC is not likely to be a suitable intervention. Incidence thresholds, based on cost per case and per disability-adjusted life year averted, indicated that SMC might still be worthwhile in some areas, particularly in southern Tanzania, Malawi and northern Mozambique, but this needs further investigation. For SMC to be deployed in southern and eastern Africa, an alternative to the SP-AQ combination would be needed owing to high levels of SP resistance [15] . The difficulties in estimating the malaria burden in Africa accurately are well recognized [3] , [9] , [11] , [16] , [17] , [18] . Our emphasis was to derive a plausible and conservative estimate of the malaria burden using transparent methods, rather than aiming to produce an alternative estimate to those provided by others. However, burden estimates based on different approaches showed broadly consistent figures. The estimates using the MAP prevalence–incidence function were lowest, but it is clear from comparison with data from SMC sites that these are likely to be an underestimate as the function relates prevalence in children to all-age incidence rather than incidence in children under 5 years of age. Furthermore, the estimates produced using the WMR method were similar to those derived using a prevalence–incidence function fitted specifically to incidence data on children under 5 years of age (Griffin J., personal communication). Our estimate of the impact of SMC on mortality is simplistic, assuming that a reduction in malaria cases would be accompanied by a proportional reduction in malaria deaths. However, our estimates of impact do not include the reductions in indirect mortality that may result from better control of malaria. Some of the areas with the highest malaria burden in all of Africa lie within the parts of the Sahel and sub-Sahel, which we have identified as being suitable for SMC [2] . Deployment of SMC in these areas would be expected to be highly cost effective on the basis of the high malaria incidence per child each year. The coverage and efficacy that would be achieved, if SMC was to be implemented as a large-scale public health measure, is not yet known, but high coverage has been achieved by community-based health workers [7] , and efficacy should remain high where SP and AQ resistance levels remain low or moderate. Furthermore, our analysis suggests that even with moderate levels of coverage, the deployment of SMC could have a significant public health impact. The epidemiological and geographical situations in which SMC is likely to be useful can be defined on the basis of epidemiological data and surrogate measures of seasonality in malaria transmission. A simple algorithm could be developed to help policy makers to decide whether the malaria incidence in their country, or certain regions within their country, was sufficiently seasonal for the deployment of SMC. The algorithm could also indicate the potential impact of implementation of SMC with different levels of efficacy and coverage. Although the burden of malaria in the areas where SMC could be deployed is uncertain, it is likely to be considerable. Our analyses suggest that even where other effective malaria control tools, such as insecticide-treated nets (ITNs), indoor residual spraying of insecticides (IRS) and partially effective malaria vaccines are deployed, SMC could potentially avert a very large number of malaria episodes and many thousands of unnecessary deaths in several countries where malaria is currently not adequately controlled. Defining SMC seasonality We performed a literature review to identify studies reporting incidence of parasitologically confirmed clinical malaria and/or severe malaria for 12 consecutive months. Sources of data used included published monthly malaria incidence data obtained from a systematic review conducted in 2005 (refs 12 , 19 ), surveillance data and an additional systematic review undertaken in 2010, including contact with authors. Search criteria and further details are included in Supplementary Methods , Supplementary Table S5 and Supplementary Fig. S1 . Locations of the sites are shown in Supplementary Figs S2,3 . A previous analysis indicated that ≥75% of malaria incidence occurring within 6 consecutive months provided a useful definition of 'marked seasonality' [12] . Most of the evidence for the efficacy and safety of SMC relates to monthly delivery over a 3-month period, which provided protection during a transmission peak of 3-to-4 months. We therefore explored different definitions of the degree of seasonality based on the maximum percentage of the total annual malaria burden occurring within any consecutive four-month period. Three definitions were considered: at least 75% (definition A), 60% (definition B) and 50% (definition C) of the total annual incidence of malaria within four consecutive months. Identifying spatial predictors of SMC areas To characterize seasonality in malaria incidence outside the areas, for which epidemiological data were available, we explored whether rainfall patterns, estimated from a combination of satellite imagery and rain gauge data [20] , could be used as a predictor of the degree of seasonality in incidence. Daily accumulated rainfall data were available for a grid of 0.1 degree×0.1 degree resolution, with data missing for only 2 days since November 2000. We used data from 2002 to 2009 and aggregated the daily time series to time series using 64 points per year. Fourier analyses were undertaken to capture the average seasonality over this time period. Each site identified by our review was geo-referenced and site-specific rainfall data obtained. For each location of interest, we selected the pixel closest to the given longitude/latitude. The percentage (in 5% intervals) of the annual total rainfall occurring in a range of different consecutive periods (ranging from 2 to 6 months) was then calculated to create a set of potential indicators of seasonality. The sensitivity and specificity of each indicator variable as a predictor of the degree of seasonality in malaria incidence was calculated to create receiver operating characteristic (ROC) curves using Stata 11 software (College Station, Texas, USA). The best predictor of seasonality in malaria incidence was then used to map areas suitable for SMC across Africa using the 0.1 degree×0.1 degree grid of rainfall data. For each pixel, the seasonality in rainfall was calculated by assessing the maximum percentage of the total annual rainfall occurring in a period of consecutive months. Pixels meeting the criterion specified by the best indicator variable were considered as potentially suitable for SMC. To further improve the biological plausibility of the spatial mapping of SMC areas, we merged the map produced by seasonality in rainfall with spatial malaria endemicity estimates produced by MAP for 2010 (ref. 21 ), restricting the area mapped by seasonality in rainfall to include only areas with stable P . falciparum transmission (annual incidence of P. falciparum infections >0.1 per 1,000 population per annum). Estimating the population and burden in SMC areas The total population at risk in the areas identified by the approach described above was derived from LandScan 2007 population estimates [22] . Population estimates were aggregated within first administrative level and then by country, and scaled to 2010 by applying national growth rates from UN projections [23] . We estimated the number of children under 5 years of age using UN demographic information for each country [23] and the percentage living in urban/rural areas based on a population density threshold [24] . For full details, see Supplementary Methods . Malaria incidence in children under 5 years of age in SMC areas was estimated using two published methods ( Table 5 ). The first follows the approach used in the 2008 WMR for countries where estimates of malaria incidence could not be made from routinely reported data [9] , [25] . Fixed age-specific incidence rates were used according to the level of malaria risk as defined by the Mapping Malaria Risk in Africa map, and in high-transmission areas, incidence estimates were halved for populations living in urban areas [13] . To retain transparency, incidence estimates were not reduced further to account for coverage of other malaria control tools; the possible impact of interventions such as ITNs and IRS are considered in a sensitivity analysis. The second method used a published function relating annual all-age incidence to prevalence of parasitaemia in children 2–10 years of age [10] . We applied the central estimate of this function to the MAP prevalence data to estimate incidence ( Fig. 4 ). The effect of urban residence is incorporated in the prevalence estimates [2] and is, therefore, implicitly accounted for. By comparison with observed incidence/prevalence observations made in SMC studies, this relationship is likely to result in a conservative estimate of the incidence of malaria in children under 5 years of age during the transmission peak for a given prevalence ( Fig. 4 ). Table 5 Summary of methods used to estimate incidence of clinical episodes of malaria and malaria mortality. Full size table Figure 4: Prevalence and incidence of malaria detected in SMC studies and the MAP prevalence-incidence relationship. Data points show observed incidence against end of season prevalence from control or placebo groups in IPTc studies from Niakhar, Senegal [30] ; Hohoe, Ghana [31] ; Kambila, Mali [32] ; Bobo-Dioulasso, Burkina Faso (Zongo I., personal communication); Kati, Mali [27] and Boussé, Burkina Faso [26] . Data points show malaria incidence defined as fever plus parasitaemia of any density or with a local defined parasite density cutoff, and are shown against the left vertical axis. All studies included children under 5 years of age, with the exception of the Kambila IPTc study, which included children under 10 years of age. For the Kambila IPTc study (Mali) the prevalence estimate at the start of the transmission season (92/262, 35.1%) was used rather than that measured at the end of the transmission season, as this was based on relatively small numbers (8/54, 15%). The curve shows the fitted relationship between all age incidence per annum and prevalence in children 2–10 years of age, 13 and is shown against the right vertical axis. Dashed lines show the upper and lower limit of the incidence-prevalence relationship defined by the IPTc data points. Full size image The mortality burden in SMC areas was also estimated by two approaches ( Table 5 ). Method one assumes a fixed CFR of 4.5 deaths per 1,000 malaria cases (0.45%), the central estimate for areas where malaria morbidity is routinely reported [9] . This fixed CFR was applied to incidence estimates derived using both the WMR method and the MAP incidence–prevalence function. We also explored a higher case fatality rate of 10 per 1,000 (that is, 1% fatality rate). Method 2 uses the approach of Rowe et al ., applying a fixed mortality rate to populations at risk rather than to malaria cases [11] . For simplicity, we did not amend our estimates to take account of the relative contribution of malaria to all-cause under 5 mortality, as performed in the WMR, but this would only be expected to reduce the estimates by ~10% (ref. 9 ). The burden in SMC areas above minimum incidence thresholds Analysis of the costs of SMC delivery undertaken by the IPTc Working Group suggests that, on the basis of both costs per case averted and cost per disability-adjusted life year averted, SMC is likely to be cost-effective where malaria incidence exceeds 0.2. episodes per child during the peak transmission season, but may not be cost effective where incidence is less than 0.1 episodes per child during the transmission peak (Pitt C, Milligan P, unpublished results). The MAP incidence–prevalence relationship suggests that incidence would be at least 0.1 episodes per child per season at a prevalence of parasitaemia >8.8%, and at least 0.2 episodes per child at a prevalence >17.3%. Using these cutoffs is likely to be highly conservative because incidence in children at a given prevalence is likely to be substantially higher than all age incidence, the prediction given by the MAP function ( Fig. 4 ). These minimum prevalence thresholds were used to map a restricted SMC area, giving a conservative estimate of the population at risk and of morbidity and mortality in areas where SMC would be appropriate on the basis of sufficiently high incidence. Estimating the potential public health impact of SMC We considered the number of cases and deaths that could potentially be averted with different levels of SMC efficacy and coverage. In sites considered suitable for SMC, the median fraction of incidence occurring in the 4 consecutive months of peak transmission was 77% and the mean 75.7% ( Supplementary Table S1,2 ). We therefore assumed that, on average, 75% of the annual burden occurred in the SMC period, but also explored the impact of SMC, if 60% and 90% of annual incidence occurred in the period when SMC was given. In recent studies of SMC in Burkina Faso and Mali, protective efficacy of 3, monthly courses over a period of three-and-a-half months from the date of the first course was 70% and 82% respectively [26] , [27] . On the basis of these figures, assuming no protective effect in the two weeks after the end of the follow-up, the protective efficacy over four months would be 61% (Burkina) and 72% (Mali), a mean of 67%. We therefore assumed that a protective efficacy of 65% would be a reasonable estimate of protection provided by three courses over a 4-month peak. Four monthly courses over 4 months might provide protective efficacy of ~80%. We explored the potential range in impact of SMC by allowing for a 25 or 50% underestimate or overestimate of the malaria burden without SMC. We accounted for a possible overestimate in this way to include the burden estimate that would be expected, had we additionally adjusted for coverage of other widely used malaria control tools. ITNs and IRS would be estimated to reduce incidence by ~50% and 60%, respectively, at 100% coverage [9] , [28] . However, actual coverage of these interventions is currently far less than 100% in most African countries [29] . How to cite this article: Cairns, M. et al . Estimating the potential public health impact of seasonal malaria chemoprevention in African children. Nat. Commun. 3:881 doi: 10.1038/ncomms1879 (2012).